Continental flood basalts derived from the hydrous mantle transition zone It has previously been postulated that the Earth’s hydrous mantle transition zone may play a key role in intraplate magmatism, but no confirmatory evidence has been reported. Here we demonstrate that hydrothermally altered subducted oceanic crust was involved in generating the late Cenozoic Chifeng continental flood basalts of East Asia. This study combines oxygen isotopes with conventional geochemistry to provide evidence for an origin in the hydrous mantle transition zone. These observations lead us to propose an alternative thermochemical model, whereby slab-triggered wet upwelling produces large volumes of melt that may rise from the hydrous mantle transition zone. This model explains the lack of pre-magmatic lithospheric extension or a hotspot track and also the arc-like signatures observed in some large-scale intracontinental magmas. Deep-Earth water cycling, linked to cold subduction, slab stagnation, wet mantle upwelling and assembly/breakup of supercontinents, can potentially account for the chemical diversity of many continental flood basalts. Continental flood basalts (CFBs) form part of large igneous provinces (LIPs) erupted onto continental crust and are characterized by anomalously high rates of mantle melting, representing the largest volcanic events in Earth’s history. Such events have significant implications for understating Earth dynamics [1] , [2] and global environmental catastrophes [3] . CFBs are conventionally attributed to decompressional melting of hot mantle, driven by mantle plumes—hot upwellings originating at the core–mantle boundary [2] . However, the chemical compositions of most CFBs are dissimilar to ocean island basalts (OIBs) [4] that are associated with hot spots—the surface expressions of mantle plumes [5] . Furthermore, although CFBs are generally several hundred kilometres from plate boundaries (subduction zones), some exhibit subduction-like geochemical signatures [4] , [6] . Petrological and geochemical evidence from the Karoo [7] , Etendeka [8] , Siberian [9] and Central Atlantic LIPs [6] suggests that generation of CFBs is ultimately related to fluid/melt derived from subducted slabs. However, the question of how fluid is released from deep subducted oceanic slabs and effects or controls partial melting of the mantle in an intracontinental setting is unclear. The mantle transition zone (MTZ) has been considered to act as a gigantic water tank in deep-Earth fluid cycling [10] , [11] , [12] , [13] , [14] , [15] , [16] , [17] due to water-enriched wadsleyite and ringwoodite at depths between 410 and 660 km (refs 11 , 13 , 16 , 17 ), which can host enough water to comprise up to 2.5% of the weight of these minerals [13] , [14] . This implies that the MTZ may play a key role in terrestrial magmatism and plate tectonics [12] , [18] . As an oceanic plate descends into the upper mantle, any fluid retained within the subducting plate beyond the depths of magma generation constitutes a return flux to the Earth’s interior [15] . Subducted oceanic slabs tend to be subhorizontally deflected or flattened as ‘stagnant slabs’ above, across or below the 660-km discontinuity [11] . Hydrous phases in the MTZ would eventually decompose into anhydrous phases by releasing fluids to produce wet upwellings that pool within the MTZ [11] , [19] . However, direct observations for the water content of the MTZ are spare and mainly inferred from geophysics [16] , [17] . With the exception of a single ∼ 10 μm ringwoodite grain from one location [13] , there is no geochemical evidence that the MTZ is water rich. Thus, finding confirmatory evidence of the origin of primary mantle melts from a hydrous MTZ is an important step in understanding deep-Earth water cycling and identifying contributions from non-plume processes in the generation of CFBs. This study suggests that oxygen isotopes, 39 Ar/ 40 Ar ages, and other geochemical features of the Chifeng CFBs of East Asia are correlated with distance to the western edge of the stagnant Pacific slab within the MTZ. We demonstrate that the lavas immediately above the western edge of the stagnant Pacific slab are characterized by being oversaturated in silica, having the oldest eruptive ages, the lowest olivine δ 18 O values and possibly the highest fluid contents. The combination of clearly recycled oceanic crust-derived signatures and their correlation with the inferred position of stagnant Pacific slab within the hydrous MTZ therefore provides an important constraint on the depth of the mantle source. These observations lead us to propose an alternative thermochemical model that may be more widely applicable, whereby slab-triggered wet upwelling produces large volumes of melt that may rise from the hydrous MTZ. This model links deep-Earth water cycling, slab stagnation, wet mantle upwelling, large-scale intraplate magmatism and assembly/ breakup of supercontinents into a self-organised system. Hydration of the MTZ by stagnant Pacific slab Central–East Asia is an ideal area to study deep-Earth water recycling on a large intracontinental scale, because Cenozoic volcanic rocks in this region ( Fig. 1 ) are associated with stagnant slabs in the MTZ [20] , [21] . The subducted slab of the Pacific plate extends horizontally over a distance of 800 to >1,000 km in the MTZ at the 660-km discontinuity [11] , [21] , [22] . Such a stagnant slab has the ability to add a large amount of subducted fluid into the mantle, with the potential for subsequent triggering of wet mantle upwelling [21] , [23] , [24] , [25] . 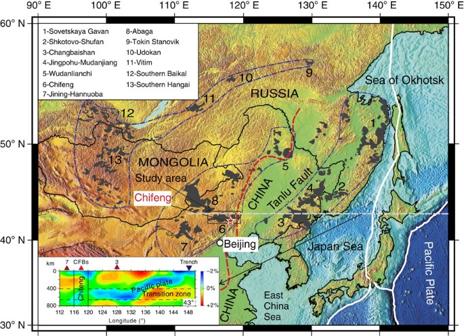Figure 1: Schematic map of the late Cenozoic intraplate volcanic province in Central–East Asia. Digital topography of Central and East Asia (original data from National Oceanic and Atmospheric Administration/National Geophysical Data Center website:http://www.ngdc.noaa.gov/mgg/image/). The dark grey colour indicates the location of late Cenozoic volcanism in Central–East Asia. The thick solid white lines represent plate boundaries. The late Cenozoic intraplate volcanic province is composed of eastern (#1−#4), central (#5−#8) and western (#10−#13) units. The eastern unit is not typically intraplate due to its close proximity to the plate boundary. The western and central units are more representative of typical intraplate volcanism. Inset figure shows the tomographic map of the inferred stagnant paleo-Pacific slab within the mantle transition zone along latitude 43° (ref22; highlighted by the grey dashed horizontally line). Numbers 3 and 7 in the inset figure represent the Changbaishan and Jining-Hannuoba volcanic rock units, respectively. The red dashed line indicates the western edge of the present-day stagnant Pacific slab21. Figure 1: Schematic map of the late Cenozoic intraplate volcanic province in Central–East Asia. Digital topography of Central and East Asia (original data from National Oceanic and Atmospheric Administration/National Geophysical Data Center website: http://www.ngdc.noaa.gov/mgg/image/ ). The dark grey colour indicates the location of late Cenozoic volcanism in Central–East Asia. The thick solid white lines represent plate boundaries. The late Cenozoic intraplate volcanic province is composed of eastern (#1−#4), central (#5−#8) and western (#10−#13) units. The eastern unit is not typically intraplate due to its close proximity to the plate boundary. The western and central units are more representative of typical intraplate volcanism. Inset figure shows the tomographic map of the inferred stagnant paleo-Pacific slab within the mantle transition zone along latitude 43° (ref 22 ; highlighted by the grey dashed horizontally line). Numbers 3 and 7 in the inset figure represent the Changbaishan and Jining-Hannuoba volcanic rock units, respectively. The red dashed line indicates the western edge of the present-day stagnant Pacific slab [21] . Full size image The Chifeng CFBs are located far from plate boundaries, but were erupted directly above the inferred edge of the Pacific stagnant slab (red dashed line in Fig. 1 ), and extend about 200 km further to the west. They were mainly (>90% volume) erupted between 23.8 and 6.1 Myr ago ( Supplementary Figs 1 and 2 ), producing 100–450-m-thick sheet-like lava flows that cover a total area of 3,000 km 2 (ref 26 ). Eighty-five samples were collected in this study from across the Chifeng CFB province to investigate the role of deep water cycling in their generation. The rocks include quartz tholeiite, olivine tholeiite and alkali basalt, all with high-sodium contents ( Supplementary Figs 3−5 ) and depletion of heavy rare earth elements ( Supplementary Fig. 5 ). All the samples show prominent positive spikes for Ba, K, Pb and Sr in the primitive mantle normalized diagram ( Supplementary Fig. 5 ), a typical characteristic of hydrated mantle melts [6] , [20] , [27] , [28] . The most striking observation is that oxygen isotopes, 39 Ar/ 40 Ar ages, and other geochemical features of the Chifeng CFBs (SiO 2 , Nb, Sm/Nd, Ce/Pb, K/Ce, Tb/Yb and Sr/Ce) are correlated with distance to the western edge of the stagnant Pacific slab ( Fig. 2 ; Supplementary Fig. 6 ). The western termination of the Pacific slab is located at ∼ 119° 30′ E (ref 22 ) (red dashed line in Fig. 1 ), with the Chifeng CFBs extending westward to around 117° E. In a westward direction, the lavas decrease in age, are depleted in silica, and have lower Sm/Nd ratios, whereas they show progressive enrichment in Nb and have higher Ce/Pb ratios. Importantly, the olivine δ 18 O values of the basalts increase westward away from the stagnant slab ( Fig. 2a ). Thus, the lavas immediately above the western edge of the stagnant Pacific slab are characterized by being oversaturated in silica, having the oldest eruptive ages, the lowest olivine δ 18 O values and possibly the highest fluid contents (high Ce/Pb, K/Ce and Sr/Ce ratios; Fig. 2a,e and Supplementary Fig. 6a,c ). 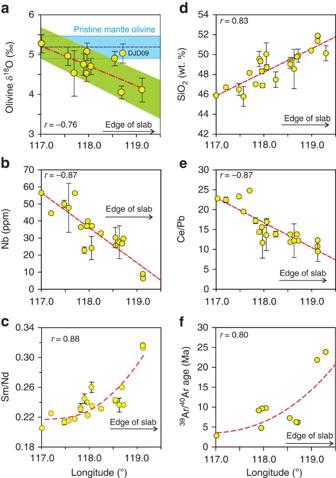Figure 2: Covariations of geochemistry as a function of eruptive longitude. (a) olivine δ18O, (b) Nb, (c) Sm/Nd, (d) SiO2, (e) Ce/Pb, and (f)39Ar/40Ar age versus longitude (°). Data points represent an average of analysed whole-rock or olivine samples from individual Chifeng CFBs (for detailed sample distribution seeSupplementary Dataset 1andSupplementary Fig. 1); error bars represent 1 s.d. for each group of lava or olivine.r, correlation coefficient. Figure 2: Covariations of geochemistry as a function of eruptive longitude. ( a ) olivine δ 18 O, ( b ) Nb, ( c ) Sm/Nd, ( d ) SiO 2 , ( e ) Ce/Pb, and ( f ) 39 Ar/ 40 Ar age versus longitude (°). Data points represent an average of analysed whole-rock or olivine samples from individual Chifeng CFBs (for detailed sample distribution see Supplementary Dataset 1 and Supplementary Fig. 1 ); error bars represent 1 s.d. for each group of lava or olivine. r , correlation coefficient. Full size image Variations in oxygen isotopes in the mantle source are ultimately related to surface water–rock interaction [29] , [30] , [31] . The oxygen isotopes of primary melts are therefore sensitive to contributions from hydrothermally altered recycled components. Partial melts of unaltered mantle peridotites record a relatively uniform value of δ 18 O olivine =5.18±0.28‰, corresponding to δ 18 O whole-rock =5.5±0.2‰ (refs 29 , 31 ). In contrast, melts of subducted sediments and the upper oceanic crust display higher δ 18 O values (≥7‰), whereas melts of subducted lower oceanic crust and altered ultramafic rocks from deeper in the ocean lithosphere are characterized by lower δ 18 O values (mostly ranging from 5‰ to 3‰) [30] . Thus, oxygen isotopes are crucial for identifying any contribution from the stagnant Pacific slab in generating the Chifeng CFBs. The olivine oxygen isotope compositions of the Chifeng CFBs reveal three prominent features: (1) a wide range of δ 18 O values varying from 3.0‰ to 5.8‰ ( Fig. 2a ; Supplementary Figs 7 and 8 ), which plot significantly beyond the range of pristine upper mantle olivine (5.18±0.28‰); (2) significant depletion of 18 O (370 of 478 total analyses have δ 18 O values <5.18‰), varying from +3‰ to 5‰, similar to those of hydrothermally altered gabbros [30] ; and (3) systematic spatial variation of average olivine δ 18 O values that are tightly correlated with eruptive site (highlighted by green band in Fig. 2a ). Because the above-mentioned features are tightly correlated with the position of the stagnant paleo-Pacific slab within the MTZ, this implies that slab stagnation, dehydration and wet upwelling may have played an important role in the generation of the Chifeng CFBs. Differentiation of the Chifeng CFBs is dominated by olivine and clinopyroxene fractionation ( Supplementary Fig. 9 ). Crystallization of olivine will increase both the silica content [32] and the δ 18 O 29 value in differentiated magmas and thus would generate positive δ 18 O-SiO 2 and negative δ 18 O-Fo correlations, respectively. This is in stark contrast with our observations ( Fig. 3a,c ). Crustal materials are generally characterized by high SiO 2 contents and high La/Sm, but low Sm/Nd, ratios, whereas asthenospheric mantle-derived melts generally have typical mantle oxygen isotopes (olivine δ 18 O of 5.18±0.28‰), lower La/Sm and higher Sm/Nd ratios compared with crustal materials. Thus, if the low δ 18 O signatures were produced by contamination of asthenospheric mantle melts by crustal materials, the δ 18 O values should positively correlate with SiO 2 and Sm/Nd ( Fig. 3a,b ) and negatively correlate with La/Sm ( Fig. 4b ). Such predicted crustal contamination trends are in distinct contrast with the observations. Furthermore, the negative SiO 2 -La/Sm and positive SiO 2 -Sm/Nd correlations are also inconsistent with predicted crustal contamination trends ( Fig. 5c,f ). Thus, contributions from assimilation and fractional crystallization processes in producing the trends observed in Figs 2 , 3 , 4 can be excluded. In summary, the correlations between olivine δ 18 O and other geochemical parameters reflect the nature of the primary melts and their source region. 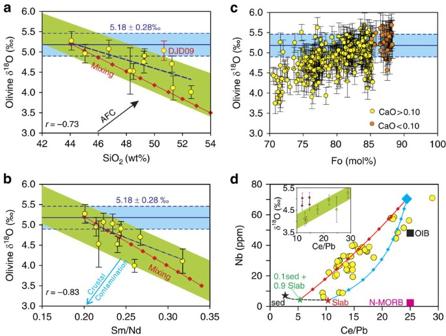Figure 3: Correlation of olivine oxygen isotopes and corresponding whole-rock major trace elements. Covariation of high-field-strength elements (HFSEs, for example, Nb) and fluid sensitive trace element ratio (Ce/Pb). Pristine upper mantle olivine oxygen isotope composition31is also shown. Mixing model endmembers inaandbare δ18O=+5.2‰ and +3.5‰, SiO2=44 and 54 wt%, Sm/Nd=0.2 and 0.34, Nb=70.4 and 4.4 p.p.m. (0.1 recycled sediment+0.9 recycled slab), and Ce/Pb=24.4 ((oceanic-island basalts (OIB)-type melt, blue diamond ind) and 5.3 (0.1 recycled sediment+0.9 recycled slab)66, respectively. The average values of alkalic OIB67and normal mid-ocean ridge basalts (N-MORB)67are also shown. AFC, assimilation fractional crystallization; sed, sediment; Fo, forsterite content of olivine inc. Solid red lines with small diamonds represent the mixing of two endmembers. Each diamond on the mixing curves represents a 10% increment of end-member melts. The detailed chemical compositions of analysed olivine are presented inSupplementary Fig. 13. Figure 3: Correlation of olivine oxygen isotopes and corresponding whole-rock major trace elements. Covariation of high-field-strength elements (HFSEs, for example, Nb) and fluid sensitive trace element ratio (Ce/Pb). Pristine upper mantle olivine oxygen isotope composition [31] is also shown. Mixing model endmembers in a and b are δ 18 O=+5.2‰ and +3.5‰, SiO 2 =44 and 54 wt%, Sm/Nd=0.2 and 0.34, Nb=70.4 and 4.4 p.p.m. (0.1 recycled sediment+0.9 recycled slab), and Ce/Pb=24.4 ((oceanic-island basalts (OIB)-type melt, blue diamond in d ) and 5.3 (0.1 recycled sediment+0.9 recycled slab) [66] , respectively. The average values of alkalic OIB [67] and normal mid-ocean ridge basalts (N-MORB) [67] are also shown. AFC, assimilation fractional crystallization; sed, sediment; Fo, forsterite content of olivine in c . Solid red lines with small diamonds represent the mixing of two endmembers. Each diamond on the mixing curves represents a 10% increment of end-member melts. The detailed chemical compositions of analysed olivine are presented in Supplementary Fig. 13 . 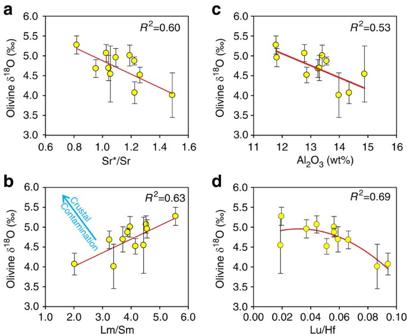Figure 4: Correlation between average oxygen isotope values and major trace elements. δ18O signatures versus (a) Sr*/Sr, (b) La/Sm, (c) Al2O3and (d) Lu/Hf. Sr*/Sr=2 × SrN/(CeN+NdN), where subscriptNindicates primitive mantle67normalized values. Because crustal materials are characterized by high La/Sm ratios, if the low δ18O signatures resulted from crustal contamination of normal asthenospheric mantle melts, a negative δ18O-La/Sm trend is expected as highlighted by the blue line with arrow inb, whereas a positive δ18O-La/Sm correlation is observed. This implies that the low δ18O signature is a primary feature of the melts. Full size image Figure 4: Correlation between average oxygen isotope values and major trace elements. δ 18 O signatures versus ( a ) Sr*/Sr, ( b ) La/Sm, ( c ) Al 2 O 3 and ( d ) Lu/Hf. Sr*/Sr=2 × Sr N /(Ce N + N d N ), where subscript N indicates primitive mantle [67] normalized values. Because crustal materials are characterized by high La/Sm ratios, if the low δ 18 O signatures resulted from crustal contamination of normal asthenospheric mantle melts, a negative δ 18 O-La/Sm trend is expected as highlighted by the blue line with arrow in b , whereas a positive δ 18 O-La/Sm correlation is observed. This implies that the low δ 18 O signature is a primary feature of the melts. 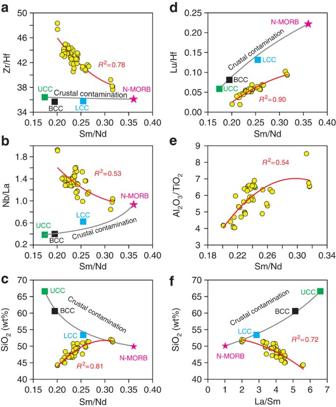Figure 5: Whole-rock geochemical covariation diagrams of the Chifeng CFBs. (a) Zr/Hf, (b) Nb/La, (c) SiO2, (d) Lu/Hf, and (e) Al2O3/TiO2versus Sm/Nd, and (f) SiO2versus La/Sm. Continental crustal materials68and normal mid-ocean ridge basalt (N-MORB)67are also shown. The contamination of asthenospheric mantle melts (N-MORB) by crustal materials, such as UCC, would result in increasing SiO2and La/Sm, but decreasing Sm/Nd in the evolved magmas, producing a positive SiO2-La/Sm, and a negative SiO2-Sm/Nd. These predicted crustal contamination trends are inconsistent with the trends observed in the Chifeng CFBs incandf. These trends demonstrate that the effects of crustal contamination can be ignored. BCC, bulk continental crust; LCC, lower continental crust; UCC, upper continental crust. Full size image Figure 5: Whole-rock geochemical covariation diagrams of the Chifeng CFBs. ( a ) Zr/Hf, ( b ) Nb/La, ( c ) SiO 2 , ( d ) Lu/Hf, and ( e ) Al 2 O 3 /TiO 2 versus Sm/Nd, and ( f ) SiO 2 versus La/Sm. Continental crustal materials [68] and normal mid-ocean ridge basalt (N-MORB) [67] are also shown. The contamination of asthenospheric mantle melts (N-MORB) by crustal materials, such as UCC, would result in increasing SiO 2 and La/Sm, but decreasing Sm/Nd in the evolved magmas, producing a positive SiO 2 -La/Sm, and a negative SiO 2 -Sm/Nd. These predicted crustal contamination trends are inconsistent with the trends observed in the Chifeng CFBs in c and f . These trends demonstrate that the effects of crustal contamination can be ignored. BCC, bulk continental crust; LCC, lower continental crust; UCC, upper continental crust. Full size image The effect of the degree of partial melting on trace element ratios of Sm/Nd, Nb/La, La/Sm and Lu/Hf at low to moderate melting fractions (0.1–0.3; Supplementary Fig. 10 ) is insignificant compared with the large variation of these ratios in the Chifeng CFBs. Thus, by excluding crustal contamination, the correlations as shown in Fig. 5 clearly suggest two end-member melts were involved in the generation of the Chifeng CFBs. The correlations in Figs 2 , 3 , 4 , 5 and Supplementary Figs 11 and 12 show that one end-member melt has an enriched OIB-like incompatible element composition, pristine upper mantle-like olivine δ 18 O values (5.18±0.28‰,) and low silica content (44%). After correction for olivine fractional crystallization by adjusting to equilibrate with Fo 90 (ref. 32 ), the OIB-like end-member melt has a chemical composition similar to that of the incipient partial melt of garnet peridotite [33] , with SiO 2 =44−46 wt%, TiO 2 =2.0−2.5 wt%, Al 2 O 3 =9.4−10 wt%, MgO=17 wt% and FeO total =10−11 wt%; Sm/Nd=0.20, Zr/Hf≥44, Nb/La≥1.4, Lu/Hf≤0.04, Al 2 O 3 /TiO 2 =4–5 and La/Sm≥4.0. The evidence from low 3 He/ 4 He ratios shows that they are similar to melts generated in the shallow mantle, but significantly lower than those generated in the primordial lower mantle [28] . The lack of lower mantle-rooted low-velocity seismic structure [21] , the alkalic nature of the dominant phase and no evidence for pre-eruption uplift [34] argue strongly against a deep plume origin for the OIB-like end-member melt [35] . The large-scale doming in the Hangai–Hövsgöl region of central Mongolia has been cited as key evidence for the presence of a mantle plume below Central Asia in the late Cenozoic [36] . However, a combined gravity- and topography-based geophysical investigation [37] demonstrated that a high-heat-flux mantle plume was unlikely to be involved because upper mantle dynamics are in reasonable agreement with the gravity, tomography, volcanic and xenolith data from the area. Recent geochemical and petrological studies [35] , [38] have demonstrated that an OIB-like enriched mantle component can form within the upper part of the mantle by enrichment with fluid or melt released from depth, possibly originating from the MTZ as we propose. The other end-member melt is characterized by low olivine δ 18 O values (3–4‰), high silica ( Fig. 3a ), depleted incompatible trace element compositions ( Figs 2c and 3b ) and subduction slab-like Ce/Pb ratios ( Fig. 3d ). Furthermore, the depletion of 18 O is coupled with depletion in high-field-strength elements (for example, Nb; Fig. 2c ) and other incompatible elements, as evidenced by decreasing La/Sm ratios ( Fig. 4b ). More importantly, the low δ 18 O end-member melt also has characteristics of melts typical of recycled oceanic crust that is dominated by gabbroic components, such as high-positive Sr anomalies ( Fig. 4a ), high Al 2 O 3 ( Fig. 4c ) and SiO 2 ( Fig. 3a ) contents, and high Fe/Mn ( Supplementary Fig. 8f ), Sm/Nd ( Fig. 3b ) and Lu/Hf ( Fig. 4d ) ratios, but low La/Sm ( Fig. 4b ) and Tb/Yb ( Supplementary Fig. 6b ) ratios. This is confirmed by the studies of olivine-hosted melt inclusions [39] from the south-eastern extremity of the Chifeng CFBs (119° 15′ E) erupted directly above the western edge of the stagnant Pacific slab. The melt inclusion data imply that these CFBs were mainly derived from an olivine-free pyroxenite-dominated source with high water content (>450 p.p.m.). These observations show that the low δ 18 O end-member melt most likely originated from hydrothermally altered oceanic gabbros [30] , [32] . Furthermore, from the systematic regional trend presented in Fig. 2 , hydrothermally altered oceanic gabbro was most likely present in the stagnant Pacific slab. Thus, the combination of clearly recycled oceanic gabbro-derived signatures and their correlation with the inferred position of stagnant Pacific slab within the hydrous MTZ provides an indirect, but important, constraint on the depth of the mantle source. For the Chifeng CFBs, the hydrous melts considered to have originated in the MTZ do not record any high δ 18 O values (>6‰). This new finding implies that water (possibly including other fluid phases) was transported into the MTZ in hydrothermally altered gabbros and possibly ultramafic rocks from the interior part of the subducted oceanic lithosphere. In contrast, the upper part of the subducted slab that would have higher δ 18 O values most likely underwent breakdown during the subduction process and may have generated high δ 18 O fluid via arc or back arc volcanism in the subduction channel. This is perhaps why high δ 18 O (>6‰) samples have not been identified in this study. Another possibility is that any high δ 18 O signatures would be diluted by low δ 18 O components, implying that the upper part of the subducted slab may play only a minor role in deep-Earth water cycling, at least in this region. In summary, the source of the CFBs is dominated by two end-member reservoirs: the stagnant Pacific slab and fertile peridotite. Mixing of melts from these two end-members can explain the major element, incompatible trace element, and oxygen isotope compositions of the Chifeng CFBs ( Fig. 3a,b,d ). The two-end-member mixing calculation shows that the source of low Ce/Pb lavas may also contain minor subducted sediments ( Fig. 3d ; Supplementary Figs 11 and 12 ). This is consistent with the coexistence of low Ce/Pb and normal olivine δ 18 O values ( ∼ 5.0‰) in individual samples. Direct or indirect contribution from stagnant slabs therefore significantly affects the upper mantle thermochemical state and has played an important role in generating the Chifeng CFBs [23] , [40] . MTZ wet upwellings produce the Chifeng CFBs These observations lead us to propose an alternative model for the Chifeng CFBs, whereby slab-triggered wet upwelling and upward percolation/hydration, which originated at the MTZ, produced large volumes of melt ( Fig. 6 ). The slow kinetics of the pyroxene–garnet transformation [41] and slab viscosity [42] within the MTZ enables the Pacific slab to reside for a long time in this zone (over 10 8 year) and hence lose water by dehydration reactions within the MTZ [11] . Because feedbacks between trench backward migration and slab deformation are integrated during the slab stagnation [42] , the declining rate of Pacific-Eurasia convergence from a late Cretaceous convergence rate of 120–140 mm year to a minimum in the Eocene of 30–40 mm year [43] may also have contributed to the Pacific slab stagnation. After completion of the pyroxene–garnet transformation [41] , the stagnant Pacific slab is likely to eventually fall into the lower mantle (slab avalanche) and release most of its water by dehydration melting when it penetrates the 660-km discontinuity [19] . The viscosity reduction due to slow grain growth may also induce slab penetration [42] . Combining geophysical and experimental studies has therefore demonstrated the presence of extensive dehydration within the MTZ beneath this region [25] . Experiments [44] and seismic investigations [45] indicate that hydrous melt or supercritical fluid is gravitationally stable atop the 410-km discontinuity and may possibly spread laterally. The density contrast between melts and surrounding solids determines the direction of material transport in the Earth and therefore the density of silicate melts plays a very important role in controlling the chemical differentiation of the Earth [46] , [47] , [48] , [49] , [50] . In this model, the density contrast between hydrous melts and coexisting minerals is a critical parameter that affects hydrous melting and consequent upwelling. Hydrous melt is denser than the associated minerals if the water content is low, whereas when the water contents increase to higher than the threshold values, the hydrous melts will be buoyant [50] . This aspect has been investigated [48] , [49] and it is confirmed that a hydrous melt formed at relatively low temperatures will be buoyant because the melt should have a large water content, but that a hydrous melt formed at high temperature will be denser. Thus, large-scale wet upwelling may be caused by a combination of slab avalanches and the positive buoyancy generated by accumulation of less-dense fluid phases. The wet upwellings will fertilize the shallow mantle (highlighted by yellow colour in Fig. 6 ) and decrease its solidus temperature, resulting in large-scale partial melting [51] . The temporal-spatial distribution of the Chifeng CFBs may thus be controlled by variations in slab stagnation and its final penetration of the 660-km discontinuity into the lower mantle. 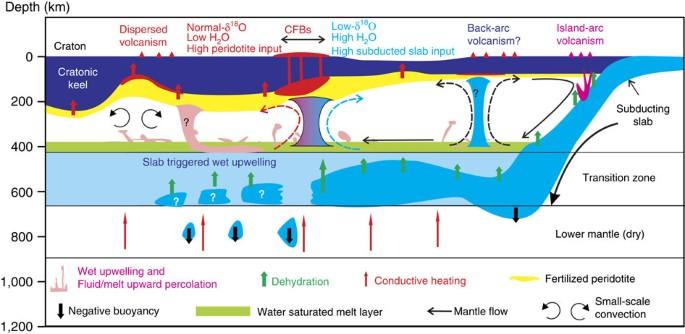Figure 6: Effects of slab stagnation and water cycling on the upper mantle thermochemical state. Water cycling refers to wet upwelling, upward percolation and refertilization. This model is mainly based on the strong spatial correlation of geochemical features with distance of eruptive lavas relative to the edge of the stagnant slab. This is based on water partitioning in the Earth’s mantle18, behaviour of slab-triggered wet upwelling and upward percolation23,40, hydrous mantle melting51, the mantle wedge model21, and upwelling from the hydrated mantle transition zone24. Figure 6: Effects of slab stagnation and water cycling on the upper mantle thermochemical state. Water cycling refers to wet upwelling, upward percolation and refertilization. This model is mainly based on the strong spatial correlation of geochemical features with distance of eruptive lavas relative to the edge of the stagnant slab. This is based on water partitioning in the Earth’s mantle [18] , behaviour of slab-triggered wet upwelling and upward percolation [23] , [40] , hydrous mantle melting [51] , the mantle wedge model [21] , and upwelling from the hydrated mantle transition zone [24] . Full size image Initial subduction of the Pacific oceanic plate under this part of Asia was inferred to take place at 130−120 Myr ago by integrating the drift history of the Pacific plate with tectonic evolution and gold mineralization in eastern China [52] . Combining the temporal distribution of volcanism and calculating the cumulative amount of total subduction within the MTZ with geophysical tomography in this region shows that collapse of stagnant slabs may have started about 25 Myr ago [12] , which coincides with the onset of eruption of the Chifeng CFBs (ca. 24 Myr ago; this study). Furthermore, because the completion of the pyroxene–garnet transformation within the MTZ will take ∼ 100 Myr ago [41] , the age of the stagnant Pacific slab is inferred to be ∼ 125 Myr ago, consistent with previous estimates [52] . Our study therefore leads to the proposition that a MTZ water-filtering model may have controlled water in the MTZ via stagnation of the Pacific oceanic plate. The contributions from water filtering [19] and high water solubility [18] result in hydration of the MTZ [10] , [11] , [12] . The hydrous MTZ model may also apply to CFBs associated with the breakup of supercontinents. Geological evidence shows that both the Pangea [53] and Rodinia [54] supercontinents were surrounded by circum—supercontinent subduction zones, a feature that seems to be true for other supercontinents and is likely to have important geodynamic implications [53] . Assembly of supercontinents therefore potentially leads to accumulation of a large volume of hydrated oceanic slabs within the MTZ [11] , [12] and may possibly change the mode of mantle convection [11] . The time delay of 140–150 Myr between the final assembly and initial breakup of Pangea [53] and Rodinia [54] is in good consistent with the lifespan of stagnant slabs within the MTZ constrained by slab viscosity [42] and phase transformation [41] . Such similarity may hint at a possible causal relationship between slab avalanche (and/or mantle overturn) and breakup of supercontinents. Slab avalanches within the hydrated MTZ would generate large-scale wet upwellings that hydrate the subcontinental lithospheric mantle ( Fig. 6 ), resulting in an instability of the lowest part of the continental lithosphere [55] , [56] . More importantly, hydrous basaltic melts would prefer to pond at the boundary between the lithosphere and asthenosphere [57] , [58] , providing a lubricating mechanism for speeding-up plate motion. The slab avalanche-driven upwelling and mobility of hydrous basaltic melts would hence promote the breakup of supercontinents and may in turn facilitate slab avalanches by adjusting trench motions and changing the geometry of subducted slabs [59] . Recent studies have proposed that the strictures of classical physics combined with modern seismic imaging, require that convective circulation in the upper mantle is plate driven and that the principal response to plate subduction and delamination is large, wide, slowly upwelling regions of mantle rooted within the MTZ [60] . Thus, plate- and slab avalanche-driven upwelling originating from the hydrous MTZ may have played an important role in the breakup of supercontinents and the circulation of water (and possibly other fluid phases) between Earth’s surface and the MTZ. The arc-like geochemical features of CFBs are traditionally attributed to continental lithosphere (both crust and mantle) input. The presence of strong arc-like geochemical signatures and hydrous phenocrysts in some high-magnesium basaltic rocks from the Siberia [9] and Karoo [7] LIPs show that crustal contamination cannot be the controlling factor. Detailed geochemical and isotopic analyses of basaltic rocks from the Siberia [9] , Karoo [7] and Central Atlantic [6] LIPs demonstrate that their generations involved water and possibly other fluid phases released from subducted slabs and that their source reservoirs were both isolated and hydrated over a considerable period of time. Because the hydration processes would result in instability of subcontinental lithospheric mantle [56] , hydrated subcontinental lithospheric mantle cannot remain isolated from the convective upper mantle. Geochemical studies and thermochemical modelling suggest that the massive degassing of volatiles (CO 2 and HCl) in some CFBs mostly originates from recycled crust in the deep Earth [61] . These observations show that continental lithosphere cannot be the dominant reservoir that produces the observed hydrous and arc-like geochemical characteristics of these CFBs. Thus, finding a mechanism to explain the long-term hydration and isolated nature of the mantle reservoir beneath the lithosphere is crucial for understanding the origin of CFBs. The deep-Earth cycling of water thus requires a fresh perspective to explain long-term hydration and its isolation within the mantle. For example, water and other fluid phases released from stagnant slabs carry large-ion lithophile elements such as Ba, Pb, K and Sr, and light rare earth elements (La to Nd), but are not able to carry high-field-strength elements such as Nb, Ta and Ti [9] . Long-term hydration and isolation within the MTZ therefore provide a mechanism to produce a hydrated reservoir that is characterized by both low high-field-strength and high large-ion lithophile element abundances and enriched radiogenic isotopes—a characteristic of arc-like CFBs [4] , [6] , [7] , [8] , [9] . Water-driven wet mantle will rise by its own buoyancy and melt on crossing its wet solidus beneath supercontinents. Such a water cycle, linked to cold subduction, slab stagnation and downward fluid transfer in the MTZ by water filtering, is expected to produce arc-like CFBs [4] , [6] , [7] , [8] , [9] with chemistry similar to that of island arcs, but at greater distances from the trench. These processes may account for the geochemical diversity of CFBs that makes them elementally and isotopically distinct from OIBs [4] . In this model, mantle upwelling is driven by deep-Earth water cycling rather than excess temperature, such as in a classical thermal plume model, which can cause about 0.8–1 km of broad surface uplift per 100 °C of plume excess temperature [62] . Because the wet upwelling of mantle requires no excess temperature in this model, there will be no thermal anomaly to result in pre-volcanic eruption surface uplift [62] . Also, some parts of the subducted slab may undergo dehydration melting and release water when it penetrates the 660-km discontinuity into the lower mantle [19] , whereas other subducted slab fragments may be entrapped in wet upwellings and returned to the upper mantle [10] , [51] . The latter provides a variant of the model that also accounts for the involvement of deep subducted slabs in the generation of large-scale intracontinental magmatism. In addition, numerical simulations [23] and geophysical investigations [11] , [21] , [22] have demonstrated that volcanism produced by wet upwelling of the mantle originating from a hydrated MTZ can be located between 600 and over 1,000 km from the trench. This can lead to CFB provinces being located at the margins of Precambrian cratons [1] . The evidence for a craton-accreted terrane setting is particularly well established for the Central Atlantic LIP, where Paleozoic island arcs and continental fragments were accreted onto the eastern margin of Laurentia during the assembly of Pangea [4] . Subsequently, the Central Atlantic LIP was extruded directly onto these terranes during the breakup of Pangea. The dominant arc-like, low-Ti-type basalts [4] , [9] within the Siberian LIP have also been attributed to wet upwelling, driven by dehydration of the Mongolia–Okhotsk oceanic slab at the MTZ [9] . Finally, water and other fluid phases released from the hydrated MTZ may also lead over time to melt accumulating at the lithosphere–asthenosphere boundary [57] , [58] . Accumulated melts can escape to the surface through weak zones, such as pre-existing suture zones, within the lithosphere. This explains why CFB provinces are commonly located over suture zones [1] . Accumulated hydrous melts at the LAB have the potential to behave as a lubricant to continent rifting and thus enhance the breakup of supercontinents. This means that arc-like CFBs, such as the Karoo, Central Atlantic and Siberian LIPs, were prominent in the initial breakup of Pangea. Here we emphasize that the presence of a plume that originated at the core–mantle boundary is not a necessary condition for producing arc-like CFBs, especially those associated with rifting and initial breakup of supercontinents. Whole-rock major and trace element analysis Seventy-three fresh basalts samples were collected from the Chifeng-Keshiketengqi area (119° 30′ E−117° 00′ E, 42° 00′ N−43° 20′ N; Supplementary Fig. 1 ) for major element analysis ( Supplementary Dataset 1 ), 45 of which were further analysed for whole-rock trace elements ( Supplementary Dataset 2 ). Rock samples were sawn into slabs and the central parts (>200 g) were used for bulk-rock analyses. The slabs were crushed into small fragments (<0.5 cm in diameter) in a jaw crusher before being further cleaned and reduced to powder in a corundum mill. Bulk-rock major element oxides were analysed using X-ray fluorescence (Rikagu RIX 2,100) with analytical uncertainties better than 3% for SiO 2 , Al 2 O 3 , Fe 2 O 3 , MgO, CaO, Na 2 O and K 2 O and better than 5% for TiO 2 , MnO and P 2 O 5 . Trace elements were analysed using inductively coupled plasma mass spectrometry at the Key Laboratory of Continental Dynamics, Northwest University, Xi’an, after acid digestion of samples in Teflon bombs. Repeated runs gave <3% relative standard deviation for most trace elements analysed. Mount making Eleven samples which were analysed for whole-rock major and trace elements were chosen to separate olivine grains for electron microscope chemical and in situ secondary-ion mass spectrometry (SIMS) oxygen isotope analyses ( Supplementary Dataset 3 ). The separated olivine grains were mounted together with reference San Carlos olivine (δ 18 O=5.35‰; Eiler [29] ) in the centre of epoxy resin mounts. The mounts were then ground and polished using different grain size Diamond Films to minimize any relief difference. Electron microscope analysis Chemical compositions of olivines were determined using a JEOL JXA-8,100 Superprobe at the Institute of Geology and Geophysics, Chinese Academy of Sciences (IGGCAS), Beijing. The operating conditions were: 15 kV accelerating voltage, 20 nA beam current, 3 μm beam diameter and 10 s peak counting time for most elements (30 s for Ca and Ni, 7 s for Na and 8 s for K). The data reduction was carried out using the atomic number, absorption, and characteristic fluorescence (ZAF) correction. In situ SIMS olivine oxygen isotope analysis The sample mount was gold coated and oxygen isotope compositions of olivines were analysed with a CAMECA IMS-1,280 ion microprobe at the IGGCAS. The Cs + primary beam was accelerated at 10 kV with an intensity of ca. 2 nA. The spot size was about 20 μm in diameter (10 μm beam diameter+10 μm raster). The normal incidence electron flood gun was used to compensate for sample charging during analysis. Secondary ions were extracted with a −10 kV potential. Oxygen isotopes were measured in multi-collector mode with two off-axis Faraday cups with a mass resolution of 2,500 (exit slit #1) in a circular focusing mode. Each analysis consisted of 20 cycles × 4 s counting time. Typical ion intensities of 2–4 × 10 6 counts per second obtained on the 18 O peak yielded an internal 2 σ uncertainty of better than ±0.2‰. Three unknown and two standard δ 18 O measurements were run in bracketed mode. Measured 18 O/ 16 O ratios were normalized using the Vienna Standard Mean Ocean Water composition (VSMOW, 18 O/ 16 O=0.0020052), and then corrected for instrumental mass fractionation (IMF) as follows: The unknown olivine data were corrected for IMF and calculated as a function of time within the standard blocks, to derive an average between the standard measurements at the beginning and end of each cycle. The external reproducibility of the standard (San Carlos) for δ 18 O is 0.4‰ 2 s.d., which was set as the error for individual measurements. Many studies have proved that there is no obvious matrix effect for olivine with Fo number >70 and San Carlos olivine standard (Fo=91) [63] , [64] , [65] . However, olivine with Fo number <65 has been proven to show about 0.6 permil bias IMF with San Carlos olivine as the standard [65] . Considering the unknown olivine grains have Fo number ranging from 60 to 91, we selected only grains with Fo >70 for oxygen isotope analysis. Thus, the potential matrix effect need not be considered further. 40 Ar/ 39 Ar analysis Twelve groundmass samples were dated using the step-heating 40 Ar/ 39 Ar method ( Supplementary Dataset 4 ). 40 Ar/ 39 Ar measurements were performed at the IGGCAS, Beijing. To constrain the eruption age and avoid excess argon, the groundmass grains with grain size ranging from 0.2 to 0.3 mm were purified carefully under a binocular microscope to remove the visible phenocrysts and xenocrysts. The samples were cleaned with acetone followed by further cleaning with deionized water in an ultrasonic bath for three times, each for 40 min. The cleaned samples were then dried at ∼ 100 °C for 20 min. Groundmass wafers weighing 3–16 mg, and multiple samples of the 18.6±0.4 Ma neutron fluence monitor mineral Brione muscovite, were irradiated in vacuo within a cadmium-coated quartz vial for 5 h in position H8 of the Beijing Atomic Energy Research Institute reactor (49–2). The argon isotopes were analysed on a MM5400 mass spectrometer. How to cite this article: Wang, X.-C. et al. Continental flood basalts derived from the hydrous mantle transition zone. Nat. Commun. 6:7700 doi: 10.1038/ncomms8700 (2015).